Growth of carbon nanotubes via twisted graphene nanoribbons Carbon nanotubes have long been described as rolled-up graphene sheets. It is only fairly recently observed that longitudinal cleavage of carbon nanotubes, using chemical, catalytical and electrical approaches, unzips them into thin graphene strips of various widths, the so-called graphene nanoribbons. In contrast, rolling up these flimsy ribbons into tubes in a real experiment has not been possible. Theoretical studies conducted by Kit et al . recently demonstrated the tube formation through twisting of graphene nanoribbon, an idea very different from the rolling-up postulation. Here we report the first experimental evidence of a thermally induced self-intertwining of graphene nanoribbons for the preferential synthesis of (7, 2) and (8, 1) tubes within parent-tube templates. Through the tailoring of ribbon’s width and edge, the present finding adds a radically new aspect to the understanding of carbon nanotube formation, shedding much light on not only the future chirality tuning, but also contemporary nanomaterials engineering. Attempting carbon nanotubes (CNTs) synthesis from graphene has been a captivating and yet challenging task. Although it is theoretically feasible [1] , there has been no effective experimental approach to materialize it so far. To tackle this unresolved issue, the nanotesttube chemistry [2] , in which a CNT is generally used as a container-cum-reactor [3] , [4] , is found to be promising. There are several studies devoted to the fabrication of graphene nanoribbons (GNRs) in CNTs through the confined polymerization of polycyclic aromatic hydrocarbon molecules [5] , [6] . In addition, the theoretical models proposed by Jiang et al . [7] have suggested that the GNRs residing in CNTs would form a helical conformation due to the geometric constraints imposed by an outer tube. The geometric constraints would restrict the chirality of CNTs synthesized. By carefully choosing the polycyclic aromatic hydrocarbon precursors, one can, therefore, foresee a controllable tuning of the different chiralities synthesized. With the inner-shell extraction technique developed recently [8] , precise verification of the CNTs synthesized is also possible through photoluminescence (PL) measurements [9] . Indeed, the present experiments demonstrate that the GNRs derived from perylene derivative are preferentially converted to (7, 2) and (8, 1) tubes in 1.4 nm outer tubes, providing strong evidence to the intertwining of both single and double strands of GNRs. Our present findings add a radically new aspect to the understanding of CNT formation, contributing not only to the future selective predetermined growth, but also to the novel nanomaterials engineering. Construction overview As shown in Fig. 1a , we can visualize the corresponding chiralities which can be formed from the twisting of a single/double strands of GNRs with an armchair edge of width N =5 as a typical example (a detailed definition of the GNR structure is given by Fujita et al . [10] ). 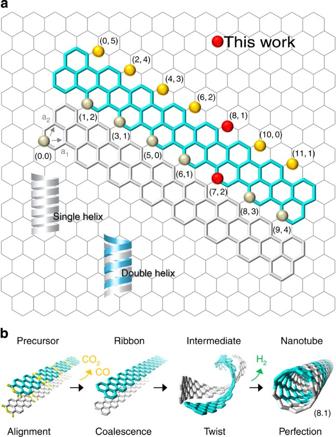Figure 1: Selective fabrication of CNTs through GNRs. (a) Map of chiral vectors showing the possible (n,m) indices obtained from the intertwining of helical perylene chains. (b) Basic steps for the synthesis of CNTs via twisted GNRs path, illustrated with a stick model of the perylene-3,4,9,10-tetracarboxylic dianhydride monomers. Blue and white, carbon; yellow, oxygen; hydrogens are omitted for simplicity. The precursors align themselves inside the CNTs. Thermal treatment results in the removal of the heteroatoms as CO and CO2. Covalent interlinking of the radical intermediates results in the extended polyaromatic chains. The subsequent twist and cyclodehydrogenation lead to the assembly of a complete tubular structure with well-defined chirality. Figure 1: Selective fabrication of CNTs through GNRs. ( a ) Map of chiral vectors showing the possible ( n , m ) indices obtained from the intertwining of helical perylene chains. ( b ) Basic steps for the synthesis of CNTs via twisted GNRs path, illustrated with a stick model of the perylene-3,4,9,10-tetracarboxylic dianhydride monomers. Blue and white, carbon; yellow, oxygen; hydrogens are omitted for simplicity. The precursors align themselves inside the CNTs. Thermal treatment results in the removal of the heteroatoms as CO and CO 2 . Covalent interlinking of the radical intermediates results in the extended polyaromatic chains. The subsequent twist and cyclodehydrogenation lead to the assembly of a complete tubular structure with well-defined chirality. Full size image The corresponding reaction mechanism is schematically depicted in Fig. 1b . It is carried out from perylene-3,4,9,10-tetracarboxylic dianhydride (PTCDA), a perylene derivative. The precursors sublime and align themselves into two linear arrays within the confined space of a host CNT. The oxygen atoms are released in the form of CO and CO 2 under mild heat treatment, yielding the radical species which subsequently polymerize into the GNRs ( Supplementary Fig. S1 ). Thermally driven helical twist of the GNRs accompanied by a cyclodehydrogenation completes the transformation into the tubular structure under vigorous annealing. Entangling of either a single- or double-helical perylene chain(s) results in the formation of tubes bearing specific chirality as predicted from the two-dimensional honeycomb map ( Fig. 1a ). Precursor-dependent inner tubes formation To confirm the proposed reaction route of PTCDA, a series of different precursors was also employed in this study, including the commonly used fullerenes (C 60 , C 70 ) and ferrocene (FeCp 2 ), and the linear polyaromatic compounds such as pentacene and picene ( Supplementary Fig. S2 ). They were first filled into the centre cavity of a parent tube, followed by a 1,200 °C-annealing to induce transformation. These newly formed inner tubes were subsequently extracted using ultrasonication [8] and further separated from the outer tube templates by density gradient ultracentrifugation (DGU) [11] , [12] ( Fig. 2a ). The procedure is described in detail in the Methods section. 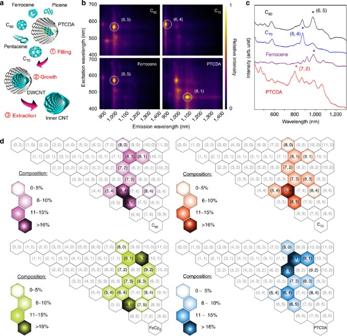Figure 2: Inner tubes grown from different precursors. (a) Schematic diagram of non-catalytic synthesis of single-wall CNTs within a parent-tube template. Precursors were first encapsulated into the interior nanospace and subsequently annealed at 1,200 °C to induce growth. Newly formed inner tubes were then extracted via sonication and further separated from the bulk outer tube templates using DGU. (b) PL contour maps of the separated inner tubes. DGU separation shows no selectivity preference towards any particular (n,m) species. (c) Optical spectra of the corresponding inner tubes synthesized. The asterisk mark (*) indicates the major (n,m) species obtained with different precursors. (d) The (n,m) chirality map showing the different species synthesized. Relative abundance is denoted by the colour gradients, computed from the respective spectral fits inc(Supplementary Fig. S6). Figure 2: Inner tubes grown from different precursors. ( a ) Schematic diagram of non-catalytic synthesis of single-wall CNTs within a parent-tube template. Precursors were first encapsulated into the interior nanospace and subsequently annealed at 1,200 °C to induce growth. Newly formed inner tubes were then extracted via sonication and further separated from the bulk outer tube templates using DGU. ( b ) PL contour maps of the separated inner tubes. DGU separation shows no selectivity preference towards any particular ( n , m ) species. ( c ) Optical spectra of the corresponding inner tubes synthesized. The asterisk mark (*) indicates the major ( n , m ) species obtained with different precursors. ( d ) The ( n , m ) chirality map showing the different species synthesized. Relative abundance is denoted by the colour gradients, computed from the respective spectral fits in c ( Supplementary Fig. S6 ). Full size image In general, the extracted inner tubes are ~40–80 nm long ( Supplementary Fig. S3 ). The corresponding optical spectra of the inner tubes retrieved are illustrated in Fig. 2b,c . The PL signals observed in Fig. 2b originate solely from the extracted inner tubes, which are fabricated from the inserted precursors. A pristine sample of the laser-ablation-synthesized parent-tube templates of 1.4±0.1 nm has no spectral contribution over the inspected range ( Supplementary Figs S4 and S5a ). Compared with the others, a distinctively different chiral distribution can be observed in the PL map of the tubes grown from the PTCDA molecules ( Fig. 2b ). A significantly intense (8, 1) signal was recorded for PTCDA, whereas C 60 , C 70 and FeCp 2 preferentially form (6, 5) or (6, 4) tubes. Absorption spectra obtained in Fig. 2c reveal that the PTCDA gives rise to not only (8, 1) tubes but also (7, 2) tubes with an S 11 excitonic transition at 802 nm [13] . The presence of (7, 2) tubes was further confirmed by using Raman spectroscopy ( Supplementary Fig. S5b ). Deconvolution of the absorption spectra between 720 and 1,200 nm in Fig. 2c ( Supplementary Fig. S6 ), the S 11 region, allows a quantitative comparison to be made on the relative abundance of contributing chiral components in each sample [14] , [15] , [16] , which is computed in Fig. 2d . In addition, to aid the characterization of metallic content composition, a series of different excitation wavelengths at 455–514 nm were employed ( Supplementary Fig. S7 ) and the overlapping M 11 , S 22 region (450–620 nm) of the absorption spectra in Fig. 2c was deconvoluted ( Supplementary Fig. S8 ). Regardless of which inner tube samples, the metallic contribution is relatively low in general as compared with the semiconducting counterparts ( Supplementary Fig. S8 ). It was found that the PTCDA-derived samples provide a majority of both (7, 2) and (8, 1) tubes, whereas the (6, 4) and (6, 5) tubes are the main species in the fullerenes- and ferrocene-derived samples, which is in good agreement with the PL maps. Most importantly, the (7, 2) and (8, 1) tubes retrieved correspond well with our expected chiralities ( Fig. 1a ), which form as a consequence of intertwining the PTCDA-derived GNR(s) inside a template CNT of 1.4 nm in diameter. We, therefore, attribute the enrichment of these two chiralities to the presence of a formation path through GNR(s) zipping, which will be discussed further in the following section. Transformation of GNRs into CNTs To analyse the observed differences, we employed Raman spectroscopy and high-resolution transmission electron microscopy (HRTEM) to obtain a better insight into the transformation process. Observations were carried out on the PTCDA-filled sample, which was annealed at a series of different temperatures as shown in Fig. 3A and Supplementary Fig. S9 . New additional peaks recorded (other than those of pristine CNTs) under two different excitation wavelengths are attributable to the successful filling of the PTCDA molecules [17] . Cross-referencing to the simulated Raman spectra of PTCDA and its oligomers, as well as to those of perylene ( Supplementary Fig. S10 ), indicates that the embedded molecules exist as a heterogeneous mixture of monomers (1,296, 1,370, 1,426 and 1,452 cm −1 at a 488 nm excitation) and dimers (1,253, 1,285 and 1,360 cm −1 at 633 nm excitation) as in that of coronene-filled CNTs discussed by Fujihara et al . [6] These encapsulated precursors aligned themselves into two linear arrays within CNTs [18] as suggested by the dark inner line contrast shown in Fig. 3B(a) . 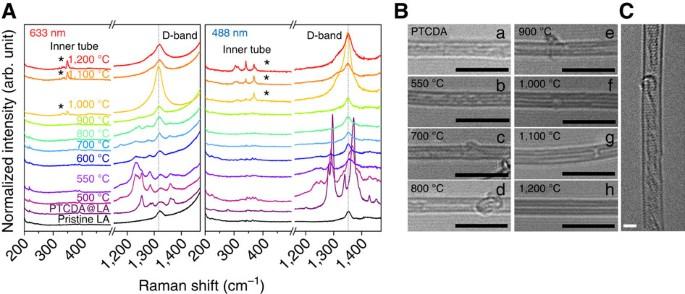Figure 3: Transformation of PTCDA molecules recorded at different annealing temperatures. (A) Raman spectra of the pristine (LA), peapod (PTCDA@LA) and the annealed samples, excited at the laser wavelengths of 633 and 488 nm. Inner tube peaks, at 300–400 cm−1, are indicated by the asterisk mark (*). The outer tube peaks of 1.4±0.1 nm, at 150–200 cm−1, are omitted (Supplementary Fig. S9). The dotted grey lines are used as a guide to the eye for the D-band feature of the CNTs. Additional spectral features other than the D-band observed in PTCDA@LA at 1,200–1,400 cm−1are attributable to that of the inserted precursors. (B)Ex situHRTEM images of the corresponding samples inA: (a) the precursor filled sample; (b–e) twisted, polymerized intermediates (to different degree); (f) confined defective tubular structure; (g, h) complete inner tubes formed. (C)Ex situAC-HRTEM image of the sample annealed at 800 °C. Several twisted loops were observed. Scale bars, 5 nm (B), 1 nm (C). Figure 3: Transformation of PTCDA molecules recorded at different annealing temperatures. ( A ) Raman spectra of the pristine (LA), peapod (PTCDA@LA) and the annealed samples, excited at the laser wavelengths of 633 and 488 nm. Inner tube peaks, at 300–400 cm −1 , are indicated by the asterisk mark (*). The outer tube peaks of 1.4±0.1 nm, at 150–200 cm −1 , are omitted ( Supplementary Fig. S9 ). The dotted grey lines are used as a guide to the eye for the D-band feature of the CNTs. Additional spectral features other than the D-band observed in PTCDA@LA at 1,200–1,400 cm −1 are attributable to that of the inserted precursors. ( B ) Ex situ HRTEM images of the corresponding samples in A : (a) the precursor filled sample; (b–e) twisted, polymerized intermediates (to different degree); (f) confined defective tubular structure; (g, h) complete inner tubes formed. ( C ) Ex situ AC-HRTEM image of the sample annealed at 800 °C. Several twisted loops were observed. Scale bars, 5 nm ( B ), 1 nm ( C ). Full size image On mild heating at 500–550 °C, new peaks arise at the vicinity of 1,230 cm −1 (633 and 488 nm), accompanied by the diminishing of peaks at 1,293 and 1,370 cm −1 (488 nm). A similar trend is displayed for the perylene-filled sample ( Supplementary Fig. S11 ), suggesting that the polymerization into longer chain fragments has occurred for both the perylene and PTCDA molecules. This is further confirmed by the simulated Raman spectra, in which a red shift of the peak (at the vicinity of 1,200–1,300 cm −1 ) towards a lower frequency is observed as the length of the oligomer increases. For PTCDAs, these extended polyaromatic chains are generated as a consequence of the endothermic elimination of oxygen atoms in forms of CO and CO 2 . This reaction produces the perylene tetraradicals that would finally merge with each other, which is similar to the synthesis of poly-peri-naphthalene [19] , [20] , [21] . Continuous elongation can be anticipated to proceed the following analogous pattern of fusion under high annealing temperatures (600–900 °C), and this explains why all the detected peaks have eventually disappeared, as the elongated GNR fragments might no longer come into resonance with the incident wavelengths. Moreover, according to the proposed geometrical structures of GNRs in CNTs by Jiang et al . [7] , we speculate that the flexible ribbons twist to adopt a versatile orientation [22] , [23] , [24] under such moderate heating condition. The hydrogen atoms along the side edges can be randomly removed as H 2 via associative desorption [25] , [26] during this stage, before the subsequent tubes formation. These helical intermediates start to exhibit a salient tubular form from 1,000 °C, as indicated by the characteristic inner tube peaks emerged at 300–400 cm −1 in the radial breathing modes (RBM) region. However, these tubes might probably have much structural defects, as suggested by a large D-band observed at 1,330 cm −1 together with transmission electron microscopy (TEM) observation of a broken line structure within the CNT ( Fig. 3B (f) ). Annealing at an elevated temperatures of 1,100–1,200 °C, however, repairs most of the defective sites (decreasing D-band), establishing perfect tubular morphology ( Fig. 3B (g) and (h) ). Coalescence of the precursor molecules induces the generation of fragments of different lengths. These neighbouring fragments of the perylene chains bump continuously into each other under heating, resulting in the entangled structures. Hydrogen atoms are constantly expelled throughout the transformation. A carbon atom may attach to another nearby carbon atom of other fragment or within similar chain by chance. This serves as an anchoring point by which the subsequent ‘zipping’ of GNRs occurs to generate CNTs ( Fig. 3C ). High temperature annealing promotes the mutual collisions as well as the H elimination, and, at the same time, provides a sufficient energy to the system to undergo an extensive bonding rearrangement. Entangling of single or double perylene-derived GNRs leads to the formation of CNTs of different chiralities as determined from the optical spectra. One may think that other polyaromatic compounds can equally form CNTs with specific chirality following a similar fusion pattern as observed in PTCDA. To obtain this information, we carried out the growth of CNTs from pentacene and picene, which consist of zigzag and armchair edge structures, respectively ( Supplementary Fig. S2 ). From the PL maps of extracted inner tubes ( Supplementary Fig. S12a ), however, it turns out that both the precursors yielded a majority of (6, 5) tubes regardless of the deferring edge structures of the reactants. Further investigation into the intermediates formed in CNTs using TEM imaging ( Supplementary Fig. S12b ) reveals that the precursors fused to give peanut-like structures, resembling those of deformed fullerenes at 550 °C. When the reaction temperature was raised to 800 °C, they grew into larger lumps converting into sausage-like structures. Complete transformation of these intermediates into the inner tubes is achieved at 1,200 °C in agreement with the Raman spectra ( Supplementary Figs S13 and S14 ) obtained. Both the reaction process and finally formed tubes show close resemblance to those of fullerenes rather than that of PTCDA. Based on the above results, we deduce that there are two possible routes for the inner CNT formation, what we call the fullerene path or GNR path, where a non-catalytic growth of CNTs occurs ( Fig. 4 ). The initial structure of the precursors does not necessarily determine the structure of the resultant CNT that is eventually produced. This is particularly obvious when all the inserted precursors, including the ball-like fullerenes (C 60 , C 70 ), pellet-like FeCp 2 and the linear polyaromatic compounds (PTCDA, pentacene and picene), lead to the formation of (6, 5) tubes to a greater or lesser degree. The key to the chirality control lies in the structural and electronic properties of the intermediates grown within CNTs. Precursors such as picene and pentacene, which lack rigid structural orientation due to their comparatively small molecular sizes, rotate freely to merge into deformed fullerene-like intermediates in the early stage [27] similar to the case of C 60 or C 70 fullerene [28] , and thus forming the thermodynamically stable (6, 5) tubes [29] . In the case of PTCDA, polymerization proceeds uniformly through the preferential elimination of anhydride ends. The radicals formed in CNTs polymerize readily into the GNR intermediates, which subsequently entangle to give a selective growth of (7, 2) or (8, 1) inner CNTs. This is different from the well-known fullerene path observed in the inner tube formation from C 60 peapods. The substantial enrichment of the preferred chiralities for the PTCDA-derived tubes is obviously insufficient to be explained only in terms of fullerene path alone. The CNTs having other chiral components present in the PTCDA fusion are considered to be the products as a result of the fullerene path fusion. This may have taken place either in CNT regions with low filling ratio, where the PTCDA molecules are not closely packed, or in a larger diameter CNTs, where there are comparatively spacious with less spatial and geometrical restrictions. 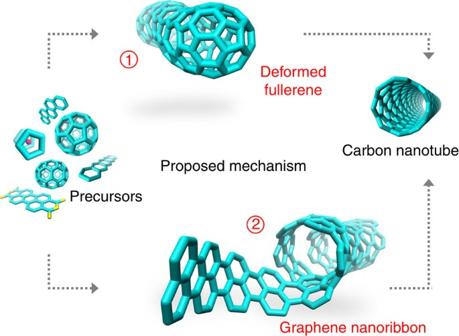Figure 4: Proposed reaction paths. We deduced that the non-catalytic transformation of the filled precursors into a well-defined CNT may proceed via two different routes of reaction, that is, (1) the conventional deformed fullerene path and (2) the twisted GNR path. Figure 4: Proposed reaction paths. We deduced that the non-catalytic transformation of the filled precursors into a well-defined CNT may proceed via two different routes of reaction, that is, (1) the conventional deformed fullerene path and (2) the twisted GNR path. Full size image The heteroatoms present in the PTCDA have also led to an improved reactivity, facilitating its polymerization into the ribbon structures and thus a higher inner tube yield. Comparing the Raman spectra of PTCDA ( Fig. 3A ) with that of perylene ( Supplementary Fig. S11 ), it is clear that the former, which has two anhydride ends attached to a perylene core ( Supplementary Fig. S1 ), polymerizes more readily to give an intense peak at 1,230 cm −1 . The CNT produced by perylene was extremely low to such an extent that the intensity of radial breathing mode peaks is almost vanishing. The chirality of the inner tubes formed is independent of the reaction time and temperature as there are no substantial changes occurring in the chirality distribution of the tubes, which are obtained with varying annealing time ( Supplementary Fig. S15 ) and temperature ( Supplementary Fig. S16 ). To obtain further information on how the singly- or doubly-joint perylene chain(s) of (7, 2) and (8, 1) could be formed, we performed quantum chemical molecular dynamics (QM/MD) simulations on the energetics and dynamics of the PTCDA peapods described above. The tendency to encapsulate either one or two PTCDA molecule(s) was evaluated by total energy calculations for ( n , 0) tubes depicted in Fig. 5a . There was no restriction set to the configuration of the embedding PTCDA molecules during the structure optimization. The binding energy, E b , was calculated in accordance with the formulas displayed in the schematics, Supplementary Fig. S17 , as reported previously by Loi et al . [30] For the CNTs of 1.4 nm in diameter used in the present study, there is no distinguishable difference observed in the energies of singly or doubly stacked structures. Although tubes having a 1.27 nm diameter may accept a doubly stacked configuration and those below 1.18 nm prefer to embed only a single molecule, they remain only a minor species in the studied CNT sample. This is consistent with the fact that no distinctive relative enhancement has been observed in the (7, 2) or (8, 1) tubes as there should be equal chances in forming a single or double GNR layer(s). 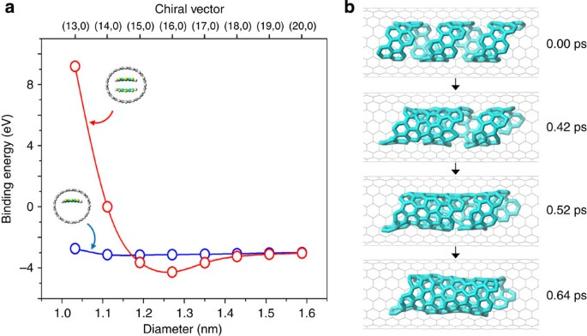Figure 5: Calculated binding energies and the snapshots of the tube-forming process. (a) Binding energy plot as a function of template tube diameter for (n, 0) peapods, with one or two PTCDA monomers. The definition of the binding energy is given inSupplementary Fig. S17. (b) Sequential transformation of the helically twisted GNR into a CNT core according to QM/MD simulations. The structure, shown in parts, exhibits an anchoring site by which the subsequent zipping of the ribbon follows (Supplementary Movie 1). Figure 5: Calculated binding energies and the snapshots of the tube-forming process. ( a ) Binding energy plot as a function of template tube diameter for ( n , 0) peapods, with one or two PTCDA monomers. The definition of the binding energy is given in Supplementary Fig. S17 . ( b ) Sequential transformation of the helically twisted GNR into a CNT core according to QM/MD simulations. The structure, shown in parts, exhibits an anchoring site by which the subsequent zipping of the ribbon follows ( Supplementary Movie 1 ). Full size image The zipping of these GNRs is even more evident from the QM/MD simulations ( Fig. 5b , Supplementary Movie 1 ). It is apparent that once the edges of a twisted GNR have come closer enough to establish a bonding formation, it acts as an initiator for zipping to proceed towards the rest of the ribbon until a complete tube is formed. Consecutive rearrangements of the pentagons, hexagons and heptagons take place gradually during the transformation. A high temperature annealing environment is needed to facilitate the process as in the experimentally observed distinct D-bands at 1,000 °C in the Raman spectra ( Fig. 3A ). A novel synthesis like this resembles a promising tool for the production of small diameter tubes with uncommon chiralities, such as (7, 2) and (8, 1), that are relatively rare in the conventional catalytic chemical vapour deposition samples. These CNTs can be potentially used as seeds for cloning of rare tubes, as reported by Liu et al . [31] Not only that, it may serve to fabricate ultrathin tubes possessing large band-gap structures, which are highly anticipated to improve the on–off ratio of CNT-based electronic devices [32] . In addition, thin CNTs produced this way are useful for solar cell application [33] , to aid the absorption of light at short wavelengths and thereby enhancing the performance. Other than that, our method has contributed a significant scientific insight towards contemporary 1D construction of novel nanomaterials. We envision a fabrication of stable DNA-like nanoribbons or even the effective manipulation of interchangeable spiral (on)—linear (off) state of the GNR@CNT in future to act as a switch, which would be very much exciting. In summary, we have demonstrated that zipping GNRs in the inner space of large-diameter CNTs is a promising route for the selective synthesis of CNTs with predetermined chiralities. A preferential growth of (7, 2) and (8, 1) tubes is achieved by using the outer tube templates of 1.4 nm in diameter. The present study poses a brand-new mechanism on the generally accepted CNTs formation occurred within the confined, minute reaction chambers, such as CNTs. Effective manipulation of the growth mechanism may lead to the creation of novel carbon nanostructures with exceptional functional properties. Inner tube formation Laser-ablation-synthesized single-wall CNTs (SWCNTs) [34] of 1.4±0.1 nm in diameter [35] were heated at 440 °C for 10 min in air to remove the capped ends before the encapsulation. 2 mg of the open-ended tubes and 10 mg PTCDA powder, (C 24 H 8 O 6 , 97%, Sigma-Aldrich), were loaded separately, degassed and sealed into the different compartments of an H-type Pyrex ampoule under a pressure of 10 −6 Torr. Vapour phase self-assembly of the PTCDA molecules into the confined hollow space of the SWCNTs took place via sublimation, where the vacuum sealed ampoule was heated in a furnace at 400 °C for 48 h. The as-prepared sample was subsequently washed with toluene (until the solution became colourless) to remove any PTCDA adsorbed on the surface of the SWCNTs. Air-dried, PTCDA-filled SWCNTs were then subjected to a high-temperature annealing at 1,200 °C for 48 h at 10 −6 Torr to induce molecular fusion. The filling of C 60 , C 70 , ferrocene (Fe(C 5 H 5 ) 2 , 98%, Sigma-Aldrich), picene (C 22 H 14 , TCI) and pentacene (C 22 H 14 , TCI) molecules was treated in a similar way described above at a lower encapsulation temperature of 300 °C except for C 60 and C 70 (600 °C) (ref. 36 ). Inner tube extraction Thermal coalescence of the confined molecules led to the generation of inner tubes within CNTs, which were then extracted using the ultrasonication approach as reported in our previous studies [8] , [9] . In brief, the annealed CNTs sample, with the capped ends reopen by heating in air at 550 °C for 10 min, was sonicated in 3.58 ml aqueous solution with 1% weight per volume (w/v) sodium deoxycholate (DOC, C 24 H 39 NaO 4 , TCI) for 20 h using an ultrasonic bath sonicator (Nanoruptor, NR-350, Cosmo Bio Co. Ltd). Separation of the extracted inner tubes from bulk The isolated inner tubes drawn from the parent tubes as a consequence of the mechanical friction caused by ultrasonication were further separated from the bulk outer CNT templates by DGU [12] . The extraction dispersant (3.58 ml) was mixed evenly with 1.42 ml of OptiPrep (60% w/v iodixanol, Sigma-Aldrich) containing 1% w/v DOC surfactants and centrifuged at 52,000 r.p.m. (163,000 g ) for 12 h at 22 °C using a swing bucket rotor (S52ST, Hitachi Koki). The resulting samples were fractionated and then characterized using optical spectroscopy. Optical characterizations Optical absorption spectra were observed by using a ultraviolet–visible spectrophotometer (V-570, JASCO). The near-infrared (NIR) fluorescence intensity was recorded as a function of excitation versus emission wavelengths for the DGU-separated samples on a spectrofluorometer (CNT-RF, Shimadzu Corp.) equipped with a liquid nitrogen-cooled InGaAs NIR detector. The excitation wavelength was set to vary in 5 nm step intervals from 400 to 700 nm, whereas the emission wavelength was detected for every 1 nm step at 850–1,400 nm. Both the emission and the excitation slit widths were set at 10 nm. Raman spectra were collected in a backscattering geometry using a single monochromator (HR-800, Horiba Jobin Yvon) equipped with a charge-coupled device (CCD) detector and an edge filter. The CNT sheets of pristine, precursor-filled and the annealed tubes were excited by a helium-neon laser at 633 nm (1.96 eV) and an argon ion laser at 488 nm (2.54 eV) unless otherwise stated. Quantitative evaluation of the extracted (n, m) composition The S 11 region of the vis-NIR absorption spectra was fitted as sums of Voigt functions of each contributing chiral species. The relative abundance of each individual species was calculated as the ratio of the area of the corresponding peak to the sum of the areas of all peaks. HRTEM observations TEM measurements were performed on a JEOL JEM-2100F operated at 80 keV at room temperature under a pressure of 10 −5 Pa. The desired sample (1 mg) was sonicated with an ultrasonic bath sonicator (30 W, VS-50R, As-One) in 1 ml of hexane solution for 15 min and drop casting onto a carbon-film-coated copper grid. TEM sample was heated at 200 °C under vacuum for 2 h to remove hexane and water moisture prior to the observation. Images were recorded on a Gatan MSC794 1 k × 1 k CCD camera with a typical exposure time of 1 s. Aberration-corrected HRTEM measurements TEM investigation was conducted using a JEOL JEM-2200MCO, equipped with a CEOS probe and image aberration correctors. The instrument was operated at an accelerating voltage of 80 keV. Images were acquired by a Gatan Ultrascan 4 k × 4 k CCD camera with 1 s acquisition times, keeping the beam current densities at ~0.01 pA nm −2 throughout. TEM samples were prepared by sonicating the 800 °C annealed peapod in 1,2-dichloroethane for 20 min and dripped onto a lacey carbon TEM grid. Raman spectra simulations The Gaussian 09 program was employed for all density functional theory calculations. Geometry optimizations and subsequent vibrational frequency analysis including Raman activity evaluations were performed with BLYP (Becke 1988 exchange+Lee, Yang, Parr correlation) functional together with 6-31G(d, p) basis set. The D 2h symmetry of the investigated PTCDA, perylene and their respective oligomers (PTCDA: C 20 n +4 H 8 n O 6 ; perylene: C 20 n H 4+8 n , n =1–4) were maintained after relaxation. Calculated harmonic vibrational frequencies were left unscaled. The Raman intensities were obtained from the computed activities following the assumption that an incident wavelength and a temperature are 1,064 nm and 25 °C, respectively. The simulated Raman spectra were generated by superposing Gaussian functions with a half-width of 3 cm −1 and heights corresponding to the calculated intensity. Binding energy calculations All the calculations were performed at the self-consistent-charge density-functional tight-binding level of theory including universal force field dispersion, using the DFTB+ program in conjunction with the standard mio-0-1 parameter set. An electronic temperature was set at 1,500 K to enhance convergence of the charge density distribution. Hydrogen-terminated ( n , 0) SWCNT systems were employed as models for the outer tube. Geometries of monomer, dimer and trimer structures were fully optimized. QM/MD simulation For QM/MD simulations, we employed the self-consistent-charge density-functional tight-binding level of theory as implemented in the DFTB+ program for the GNR subsystem. The outer (10, 10) SWCNT was included in the calculation through a classical Lennard-Jones potential taken from the universal force field dispersion, and its atomic positions were frozen throughout the simulations. The electronic temperature was set at 1,500 K to enhance convergence of the charge density distribution. A Velocity-Verlet algorithm was chosen to integrate the nuclei’s equations of motion. The canonical NVT ensemble was regulated by a Nosé–Hoover chain thermostat (chain-length=3) at a nuclear temperature of 1,500 K with 0.4 fs time steps throughout. The hydrogen atoms in the inner parts of the GNR were removed at the beginning of the simulation, which is justified by the fact that over long periods of time, the C–H bonds are being broken by high-temperature collisions and associative H 2 removal. How to cite this article: Lim, H. E. et al . Growth of carbon nanotubes via twisted graphene nanoribbons. Nat. Commun. 4:2548 doi: 10.1038/ncomms3548 (2013).